Spatial coordination between cell and nuclear shape within micropatterned endothelial cells Growing evidence suggests that cytoplasmic actin filaments are essential factors in the modulation of nuclear shape and function. However, the mechanistic understanding of the internal orchestration between cell and nuclear shape is still lacking. Here we show that orientation and deformation of the nucleus are regulated by lateral compressive forces driven by tension in central actomyosin fibres. By using a combination of micro-manipulation tools, our study reveals that tension in central stress fibres is gradually generated by anisotropic force contraction dipoles, which expand as the cell elongates and spreads. Our findings indicate that large-scale cell shape changes induce a drastic condensation of chromatin and dramatically affect cell proliferation. On the basis of these findings, we propose a simple mechanical model that quantitatively accounts for our experimental data and provides a conceptual framework for the mechanistic coordination between cell and nuclear shape. One of the most fundamental problems in tissue morphogenesis is the question of how changes in cell shape produce alterations of nuclear form and functions [1] , [2] , yet its mechanistic basis is poorly understood [3] , [4] . For instance, it is well known that the formation of new blood capillaries requires the polarization and directed migration of endothelial cells (ECs) through large cell elongations [5] , [6] , [7] , [8] , [9] . In addition, cell shape changes in ECs are commonly associated with nuclear shape remodelling [10] , [11] , [12] , [13] , which is emerging as a potential regulator of genome function [14] , [15] , [16] . To explain the link between cellular morphology and information control within living cells, Maniotis et al . [17] proposed that cell shape informations are transduced into gene expression through mechanical forces transmitted by the cytoskeleton. This assumption implies that the cytoskeleton applies forces to modulate nuclear shape and size in response to cell shape changes. Interestingly, Khatau et al . [18] have reported the presence of a dome-like actin structure, called the actin cap, that covers the top of the nucleus, and their results suggest that this structure is involved in a part of the nuclear shape deformation. More recently, a physical connection between an array of actin filaments located above the nucleus and the nuclear membrane, called transmembrane actin-associated nuclear lines, have been observed to be implicated in the intracellular localization of the nucleus [19] . Furthermore, perturbations of the intermediate filament network could alter the positioning of the nucleus in both migrating and immobile astrocytes, suggesting that cytoplasmic intermediate filaments are involved in actin-dependent positioning of the nucleus [20] . Concomitant with these recent discoveries, significant advances have been made in terms of identifying the molecular links between the nuclear envelope and the cytoplasmic filaments [21] , [22] , [23] , [24] , [25] , and new insights have been gained into the mechanistic maintenance of the nucleus [3] , [23] , [24] , [26] , [27] . Emerging evidence is now accumulating that cytoplasmic filaments are exploited by cells to govern nuclear morphology and finely tune gene expression in response to cell shape changes. However, despite the strong suspicion of the involvement of cytoskeletal actin filaments in the alteration of the intracellular force balance, no mechanical explanation exists for the adaptive remodelling of the nucleus. This problem can be tackled non-invasively by the use of adhesive islands to create a spatial environment that force single ECs to elongate, up to large-scale changes as observed in vivo [5] , [6] , [7] . We used in this study fibronectin (FN)-coated micropatterns of defined shapes and sizes to understand how changes in cell shape and spreading area (SA), which is known to be a key parameter of the cellular mechanical force balance [28] , [29] , induce cytoskeletal reorganizations that regulate the nuclear shape. In this investigation, we show that the deformation and orientation of the nucleus in response to large-scale cell shape changes are mainly controlled by lateral compressive forces and, to a lesser extent, by normal compressive forces, which are both exerted by actin filaments. We demonstrate that lateral compressive forces applied by central thick stress fibres on both sides of the nucleus regulate the nuclear shape as the cell elongates, whereas normal compressive forces are exerted by apical actin filaments to constrain the nuclear height. We show that tension in lateral stress fibres is gradually generated by anisotropic force contraction dipoles as the cell elongates and is strongly dependent on the cell SA. Our findings indicate that large-scale cell shape changes have a dramatic effect on the nuclear shape and structure, resulting in a drastic chromatin condensation and a decrease of cell proliferation. Finally, we have devised a simple physical model that relates the spatial organization and tension of central actin stress fibres to the lateral compressive forces imposed on the nucleus. This mechanical model is able to quantitatively describe the main features of nuclear shape remodelling and provides a conceptual framework for the mechanical regulation of nuclear shape and functions in response to large-scale changes in cell shape. Cell shape changes deform and orientate the nucleus To control both the cell shape index (CSI) and the SA of single ECs, we used a microcontact printing technique to pattern FN [30] and define adherent cell shapes and SAs (from 600 to 2,000 μm 2 ). We shape-engineered ECs on circular (CSI=1), square (CSI=0.79) and various rectangular (CSI=0.70, 0.50 and 0.26) adhesive micropatterns, mimicking elongated bipolar shapes observed in vivo [5] , [6] , [7] . To investigate whether large-scale changes of cell morphology could influence nuclear morphology, we assessed the CSI by differential interference contrast (DIC) microscopy and the nuclear shape index (NSI) by 4′,6-diamidino-2-phenylindole (DAPI) staining for 1,600 μm 2 shaped cells ( Fig. 1a ). 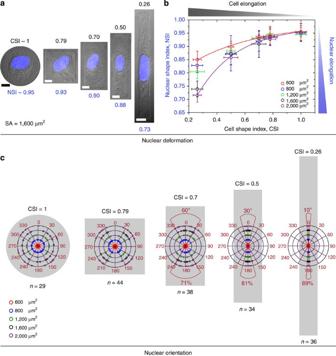Figure 1: Cell shape changes induce deformation and orientation of the nucleus. (a) DIC images of single ECs constrained on 1,600 μm2FN-coated micropatterns of various shapes (from CSI∼1 to∼0.26). The nucleus, stained in blue with DAPI and superimposed on DIC images, shows NSI ranging from 0.95 in circular-shaped cells to 0.73 in highly elongated cells. The scale bars correspond to 10 μm. (b) Evolution of NSI as a function of CSI for a wide range of SAs (from 600 to 2,000 μm2). To highlight the role of the spreading area, curves for 600 and 2,000 μm2were fitted with an asymptotic function, in red and purple, respectively. Data are given as mean±s.d. withn=15. (c) Angular graphs, superimposed on micropattern drawings in grey, show the different orientations experienced by nuclei in response to cell shape changes for various SAs (from 600 to 2,000 μm2). Data are given as mean±s.d. . As evidenced from Figure 1b , forcing the cells to spread unidirectionally on elongated patterns decrease significantly the NSI, indicating a relation between cell and nuclear shape. How cell shape may influence nuclear orientation was then investigated. Circular-shaped cells showed a random distribution of nuclear orientation spanning 360°, whereas square-shaped cells showed a preferential diagonal orientation of the nucleus, regardless of the SA ( Fig. 1c ). As the CSI decreased, nuclei became increasingly aligned with respect to the long axis of the cell, to finally reach a well-oriented state for the more pronounced elongated cell shape (CSI=0.26), characterized by a narrow angle sector (89% in a 10°-wide sector, Fig. 1c ). Taken together, these results indicate that the nucleus, initially rounded and randomly oriented in circular-shaped cells, becomes progressively deformed and anisotropically oriented as the cell elongates and spreads. Figure 1: Cell shape changes induce deformation and orientation of the nucleus. ( a ) DIC images of single ECs constrained on 1,600 μm 2 FN-coated micropatterns of various shapes (from CSI ∼ 1 to ∼ 0.26). The nucleus, stained in blue with DAPI and superimposed on DIC images, shows NSI ranging from 0.95 in circular-shaped cells to 0.73 in highly elongated cells. The scale bars correspond to 10 μm. ( b ) Evolution of NSI as a function of CSI for a wide range of SAs (from 600 to 2,000 μm 2 ). To highlight the role of the spreading area, curves for 600 and 2,000 μm 2 were fitted with an asymptotic function, in red and purple, respectively. Data are given as mean±s.d. with n =15. ( c ) Angular graphs, superimposed on micropattern drawings in grey, show the different orientations experienced by nuclei in response to cell shape changes for various SAs (from 600 to 2,000 μm 2 ). Data are given as mean±s.d. . Full size image Nuclear remodelling is mediated by the cell SA Interestingly, Figure 1b and Supplementary Figure S1 show that the nucleus was significantly more deformed when similar-shaped cells (CSI ∼ 0.26) elongated on large SAs (NSI=0.72±0.02 at 2,000 μm 2 ), suggesting that cell spreading is a key parameter of the nuclear deformation process. To further confirm this result, we fixed and stained ECs at different times during their spreading on similar elongated micropatterns ( Fig. 2a ). 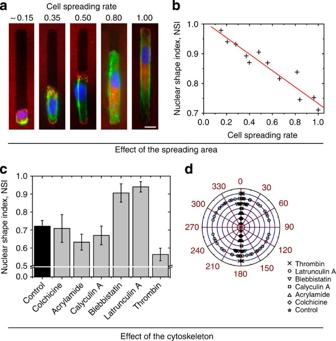Figure 2: The remodelling of the nucleus is mediated by cell spreading area and actomyosin activity. (a) Immunostained images of ECs at different spreading rates (from left to right: 0.15, 0.35, 0.50, 0.80 and 1) on elongated micropatterns with a constant surface area (1,600 μm2). The nucleus is stained in blue with DAPI, actin filaments in green with Alexa 488-phalloidin and focal adhesions in red with vinculin. The scale bar corresponds to 12 μm. (b) Evolution of the NSI of ECs as a function of their spreading rate on elongated micropatterns with a constant surface area (1,600 μm2). The red line corresponds to the best-fit linear regression. (c) Evolution of the NSI of ECs plated on 1,600 μm2elongated micropatterns (CSI=0.26) in response to various pharmacological agents. NSI for control cells is presented in black. Data are given as mean±s.d. (12≤n≤15). (d) Effect of cytoskeletal inhibitors on the angular distribution of nucleus in 1,600 μm2elongated-shaped ECs (CSI=0.26). Data are given as mean±s.d. (12≤n≤15). As shown in Figure 2b , the nucleus was rounded (NSI ∼ 0.97) when ECs started to spread and deformed linearly with increasing the spreading rate to become highly elongated (NSI ∼ 0.73 at CSI ∼ 0.26) when ECs spread completely the FN micropatterns. These results confirm our preliminary observations and underlie the importance of the cell SA in the nuclear shape remodelling process. Figure 2: The remodelling of the nucleus is mediated by cell spreading area and actomyosin activity. ( a ) Immunostained images of ECs at different spreading rates (from left to right: 0.15, 0.35, 0.50, 0.80 and 1) on elongated micropatterns with a constant surface area (1,600 μm 2 ). The nucleus is stained in blue with DAPI, actin filaments in green with Alexa 488-phalloidin and focal adhesions in red with vinculin. The scale bar corresponds to 12 μm. ( b ) Evolution of the NSI of ECs as a function of their spreading rate on elongated micropatterns with a constant surface area (1,600 μm 2 ). The red line corresponds to the best-fit linear regression. ( c ) Evolution of the NSI of ECs plated on 1,600 μm 2 elongated micropatterns (CSI=0.26) in response to various pharmacological agents. NSI for control cells is presented in black. Data are given as mean±s.d. (12≤ n≤ 15). ( d ) Effect of cytoskeletal inhibitors on the angular distribution of nucleus in 1,600 μm 2 elongated-shaped ECs (CSI=0.26). Data are given as mean±s.d. (12≤ n ≤15). Full size image Actomyosin is required for nuclear shape remodelling To gain more insight into the intracellular mechanisms that control the nuclear shape remodelling, we next consider the nuclear shape in the context of the cytoskeletal architecture. We used different pharmacological agents on 1,600 μm 2 elongated cells (CSI ∼ 0.26) to investigate the role of cytoskeletal components in determining nuclear deformation. As evidenced from Figure 2c , treatment with colchicine, which promotes microtubule depolymerization, did not significantly affect the NSI. Interestingly, alteration of intermediate filament structure with acrylamide and calyculin A allowed the NSI of elongated cells to decrease to 0.63±0.04 and 0.67±0.05, respectively ( Fig. 2c ), suggesting that intermediate filaments contribute to nuclear shape stability by balancing intracellular forces. In contrast, treatment with blebbistatin, which inhibits actomyosin contractility, and latrunculin A, which results in reduced F-actin and focal adhesion (FA) assembly, caused a significant rounding of the nucleus (NSI=0.91±0.05 and 0.94±0.03, respectively), suggesting that actomyosin activity is a key component of the nuclear deformation process. Finally, we studied the response of thrombin, a vascular permeability agent, which was observed to induce a fast retraction of ECs through increased RhoA-mediated myosin-generated contraction [31] , [32] . Remarkably, thrombin treatment resulted in larger deformation of the nucleus (NSI=0.56±0.04, Fig. 2c ), enhancing the importance of actomyosin contractility in cell shape remodelling and the critical role of the Rho pathway in determining the extent of actomyosin stress fibre [33] . We next investigated whether the disruption of these cytoskeletal components affects nuclear orientation ( Fig. 2d ). We found that nuclei of elongated cells remained significantly oriented towards the direction of long cell axis when microtubules and intermediate filaments were disrupted, indicating no involvement of these filaments in the nuclear orientation. By using blebbistatin, nuclear alignment was lower (60% within a 10°-angle window centred on the long axis of the pattern, which was set to 0°), demonstrating that myosin II activity is partially involved in nuclear orientation. After disassembling actin stress fibres with latrunculin A, we found a random orientation of the nucleus even if the cell remained elongated ( Fig. 2d and Supplementary Fig. S2 ), establishing that nuclear orientation requires stable actin filament assembly. Together, these results show that intermediate filaments provide resistance to nuclear deformation and thus help to maintain the mechanical integrity of the nucleus, whereas the mechanism governing nuclear elongation and orientation relies on actomyosin activity and actin filament organization. Stress fibre distribution in response to cell shape changes To further investigate how actomyosin activity could be converted into nuclear shape changes, we observed by laser-scanning confocal microscopy the spatial distribution of actin filaments in the central cell zone, according to the nuclear position in the cell. In circular-shaped cells, F-actin formed circular bundles resulting in the appearance of 'ring-like' F-actin structures that localized exclusively in the peripheral zone ( Fig. 3a and Supplementary Movies 1 and 2 ). In cells plated on square adhesive patterns, central actin stress fibres were observed to preferentially extent diagonally, in line with previous studies on fibroblast cells [34] . It is noteworthy that this result is consistent with the diagonal orientations of the nucleus that we observed on square-shaped cells ( Fig. 1c ). In rectangular-shaped cells, outward-curved actin stress fibres were formed along the major cell axis and localized on either side of the nucleus. As the cell became more elongated (from CSI ∼ 0.5 to ∼ 0.26), central actin stress fibres became less curved and tended to adopt a straight morphology ( Fig. 3a and Supplementary Movie 3 ). According to the observations of Khatau et al . [18] , apical F-actin network in elongated cells was observed to become oriented with respect to the long cell axis ( Supplementary Fig. S3 ). 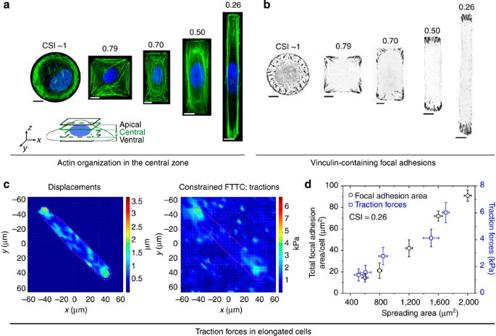Figure 3: Spatial reorganization of actin stress fibres and focal adhesions in response to cell shape changes. (a) The spatial distribution of actin filaments in the central zone (see cartoon) of ECs plated on 1,600 μm2FN-coated micropatterns was visualized by scanning laser confocal microscopy using phalloidin Alexa 488 staining after 24 h in culture. The nucleus, stained in blue with DAPI, was superimposed for clarity. The scale bars correspond to 10 μm. (b) Immunofluorescence staining for vinculin in 1,600 μm2shaped cells showing the coordinated reorganization of FAs with cell shape changes. The colour was inverted. The scale bars correspond to 10 μm. (c) Representative images of displacement and traction maps showing typical force distribution in an elongated EC (CSI∼0.26 and SA=1715 μm2). (d) Quantification of the total area of FAs per cell (in black) and tension forces (in blue) in highly elongated cells (CSI∼0.26) as a function of the SA. The area of FAs and tension forces per cell increase linearly with the SA. Data are given as mean±s.d. with 12≤n≤15 for vinculin staining and 3≤n≤7 for traction force experiments. Figure 3: Spatial reorganization of actin stress fibres and focal adhesions in response to cell shape changes. ( a ) The spatial distribution of actin filaments in the central zone (see cartoon) of ECs plated on 1,600 μm 2 FN-coated micropatterns was visualized by scanning laser confocal microscopy using phalloidin Alexa 488 staining after 24 h in culture. The nucleus, stained in blue with DAPI, was superimposed for clarity. The scale bars correspond to 10 μm. ( b ) Immunofluorescence staining for vinculin in 1,600 μm 2 shaped cells showing the coordinated reorganization of FAs with cell shape changes. The colour was inverted. The scale bars correspond to 10 μm. ( c ) Representative images of displacement and traction maps showing typical force distribution in an elongated EC (CSI ∼ 0.26 and SA=1715 μm 2 ). ( d ) Quantification of the total area of FAs per cell (in black) and tension forces (in blue) in highly elongated cells (CSI ∼ 0.26) as a function of the SA. The area of FAs and tension forces per cell increase linearly with the SA. Data are given as mean±s.d. with 12≤ n ≤15 for vinculin staining and 3≤ n ≤7 for traction force experiments. Full size image Cell shape controls FA assembly To properly understand how actomyosin filaments act on the nucleus, it would then be valuable to evaluate their tension. Previous studies have shown that local forces exerted by stress fibres in stationary cells are related to the area of FAs [28] . Therefore, we examined in a first approximation whether cell shape changes might affect spatial organization and extent of vinculin-containing FAs. After spreading on 1,600 μm 2 , shaped-cells were immunofluorescently probed for vinculin and imaged using confocal microscopy ( Fig. 3b ). Qualitatively, vinculin-containing FAs were found to be homogeneously localized along the circumference of circular-shaped cells, appeared significantly brighter and concentrated within the corner regions on square-shaped cells and finally were found to be restricted to the extremities of elongated cells ( Fig. 3b ). These observations indicate gradual but distinctive changes in the spatial distribution of vinculin-containing FAs in response to cell shape changes. After quantification of vinculin areas, we found that the total FA area formed per cell increased linearly with the extent of cell elongation from CSI ∼ 0.79 to ∼ 0.26 ( Supplementary Fig. S4 ), suggesting that the overall tension per cell increases with cell elongation. Surprisingly, disk-shaped cells were found to form a total FA area significantly larger than those measured for other cell shapes. However, due to the distribution of actin filaments in circular-shaped cells, we can reasonably consider that their nucleus were not affected by this high level of tension, as confirmed by NSI values ( Fig. 1b ) and immunostaining experiments ( Fig. 3a and Supplementary Movie 2 ). Changes in cell SA modulate traction forces To quantitatively determine the amount of tension, we next characterized the traction stress in elongated cells (CSI ∼ 0.26) by traction force microscopy (TFM) for a wide range of SAs ( Fig. 3c ). We observed that the traction stress was exclusively distributed at the edges of elongated cells ( Fig. 3c ), confirming that the traction stress is spatially correlated with adhesion areas. By examining the relationship between the total FA area and SAs for similar shaped cells (CSI ∼ 0.26), we found a linear dependence of the total FA area per cell with SAs ( Fig. 3d ). This relation indicates that FAs in elongated cells formed in proportion to the degree at which cells spread across the substrate. Interestingly, the quantification of traction stress was also found to be linearly dependent with SAs ( Fig. 3d ), indicating indirectly a dependence between tension forces and vinculin-containing FA area in elongated ECs, as suggested by Balaban et al . [28] For 1,600 μm 2 elongated cells, TFM measurements indicated a maximum tension of ∼ 5.7 kPa for a total FA area of ∼ 72 μm 2 . This result reflects an anisotropic force contraction dipole with two opposing maximum forces of ∼ 205 nN, which is consistent with the amount of forces observed in polarized fibroblasts [35] . Central actin fibres generate lateral compressive forces The next question we addressed was how tension in actin filaments acts on the nucleus in response to cell shape changes. To answer this question, we first quantified nuclear dimensions by scanning laser confocal microscopy to determine the three-dimensional relative deformations of the nucleus as a function of CSI. 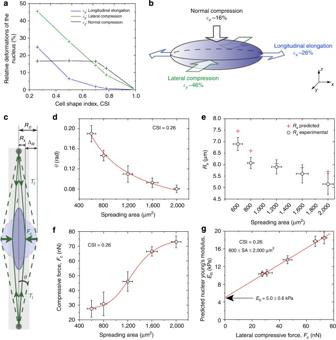Figure 4: Nuclear deformations are related to lateral compressive forces generated by central actomyosin fibres. (a) Evolution of the three-dimensional (3D) relative deformations of the nucleus as a function of the CSI (SA∼1,600 μm2). In blue: longitudinal extension (ɛx), in green: lateral compression (ɛy) and in black: normal compression (ɛz). (b) Schematic representation of the 3D relative deformations of the nucleus (CSI∼0.26 and SA∼1,600 μm2). (c) Schematic of the two-dimensional spatial organization of central actomyosin cables localized on either side of the nucleus (CSI∼0.26). On low SAs, the nucleus of elongated cells is schematically represented by a circular shape of initial radiusR0(in light blue) surrounded by two curved actomyosin fibres (dashed green lines) connected to the FA areas (dark grey circles) localized at the ends of the cell. On large SAs, the nucleus (in dark blue) is significantly squeezed and oriented by straight actin cables (green lines), which are tightened around the nucleus. Tension forces in central actin stress fibres,Tf, result in lateral compressive forces,Fcacting on both sides of the nucleus over a distance 2ΔR=2(R0−Rx). (d) Evolution of the angle of actomyosin fibres,θ, in highly elongated cells (CSI∼0.26) as a function of the SA. (e) Evolution of predicted (red crosses) and experimental (black circles) values of ΔR in highly elongated cells (CSI∼0.26) versus the SA. (f) Compressive forces,Fc, experienced by the nucleus in highly elongated ECs (CSI∼0.26) follow a sigmoidal curve as a function of the SA. (g) Predicted evolution of the nuclear Young's modulus,En, in highly elongated cells (CSI∼0.26) as a function of compressive force values reported inf. Extrapolation of the linear relation betweenEnandFcallows to estimateE0=5.0±0.6 kPa at zero-force condition. Data are given as mean±s.d. withn=12 ford,eand 12≤n≤15 forf,g. As shown in Figure 4a , during elongation the nucleus was subjected to a normal compression, ɛ z , that reached rapidly a threshold of ∼ 16%, suggesting that the nuclear height was maintained constant during large-scale cell elongations. This result is consistent with the presence of well-oriented apical actin filaments for elongated ECs ( Supplementary Fig. S3 ), whereas circular (CSI ∼ 1.0)- and squared (CSI ∼ 0.79)-shaped cells were characterized by a weak density of apical actin filaments. Interestingly, the evolution of the lateral deformation, ɛ y , showed that the nucleus underwent a lateral compression that increased linearly with decreasing CSI, to reach a maximum lateral deformation of ∼ 46%, which was threefold higher than the normal deformation. The nucleus underwent also a longitudinal elongation, ɛ x , which increased in response to cell elongation, up to ∼ 26%. This longitudinal elongation is consistent with the situation of a lateral compression applied to a deformable object with a blocked normal extension ( Fig. 4b ). Taken together, these results suggest a scenario for the nuclear shape remodelling, which is function of the cell elongation. From CSI ∼ 1 to ∼ 0.70, the nucleus experiences a quasi-homothetic deformation by balancing equivalent normal and lateral compressive forces ( Fig. 4a ), whereas from CSI ∼ 0.70 to ∼ 0.26, the nucleus extends longitudinally in response to increased lateral compressive forces and adopts an oblate spheroidal morphology ( Fig. 4b ). This indicates that the nuclear deformation of highly elongated cells is mainly induced by lateral compressive forces ( Supplementary Movie 3 ) and, to a lesser extent, by normal compressive forces. Figure 4: Nuclear deformations are related to lateral compressive forces generated by central actomyosin fibres. ( a ) Evolution of the three-dimensional (3D) relative deformations of the nucleus as a function of the CSI (SA ∼ 1,600 μm 2 ). In blue: longitudinal extension ( ɛ x ), in green: lateral compression ( ɛ y ) and in black: normal compression ( ɛ z ). ( b ) Schematic representation of the 3D relative deformations of the nucleus (CSI ∼ 0.26 and SA ∼ 1,600 μm 2 ). ( c ) Schematic of the two-dimensional spatial organization of central actomyosin cables localized on either side of the nucleus (CSI ∼ 0.26). On low SAs, the nucleus of elongated cells is schematically represented by a circular shape of initial radius R 0 (in light blue) surrounded by two curved actomyosin fibres (dashed green lines) connected to the FA areas (dark grey circles) localized at the ends of the cell. On large SAs, the nucleus (in dark blue) is significantly squeezed and oriented by straight actin cables (green lines), which are tightened around the nucleus. Tension forces in central actin stress fibres, T f , result in lateral compressive forces, F c acting on both sides of the nucleus over a distance 2Δ R =2( R 0 − R x ). ( d ) Evolution of the angle of actomyosin fibres, θ , in highly elongated cells (CSI ∼ 0.26) as a function of the SA. ( e ) Evolution of predicted (red crosses) and experimental (black circles) values of ΔR in highly elongated cells (CSI ∼ 0.26) versus the SA. ( f ) Compressive forces, F c , experienced by the nucleus in highly elongated ECs (CSI ∼ 0.26) follow a sigmoidal curve as a function of the SA. ( g ) Predicted evolution of the nuclear Young's modulus, E n , in highly elongated cells (CSI ∼ 0.26) as a function of compressive force values reported in f . Extrapolation of the linear relation between E n and F c allows to estimate E 0 =5.0±0.6 kPa at zero-force condition. Data are given as mean±s.d. with n =12 for d , e and 12≤ n ≤15 for f , g . Full size image On the basis of the relative contribution of normal and lateral compressive forces, we choose a simplifying assumption focusing only on central actin fibres. We set out to develop a two-dimensional physical model that could mechanistically describe how tension generated in lateral actomyosin filaments modulates nuclear shape. Two observations—first that curved actin stress fibres formed along the longitudinal cell direction tend to adopt a straight morphology in response to cell elongation ( Fig. 3a and Supplementary Movie 3 ), and second that tension in central actin stress fibres increases with SA ( Fig. 3d )—are central to our proposed mechanism of nuclear shape regulation. We consider the simplest situation in which the nucleus of a highly elongated cell of initial radius R 0 is symmetrically surrounded by two thick and parallel actin cables ( Fig. 4c ). Under the action of lateral compressive forces resulting from the tension in both actin cables, the nucleus is squeezed uniaxially along the x -direction over a distance 2Δ R =2( R 0 – R x ) ( Fig. 4c ). Considering the geometry of the system ( Fig. 4c ), the equilibrium between compressive forces, F c , and tension in actin stress fibres, T f , is where θ is the angle between an actin stress fibre and the vertical axis passing through its end connected to the extracellular matrix. The quantification of θ for similar elongated cells (CSI=0.26) showed an exponential decay of θ as the SA increases ( Fig. 4d ), suggesting that actin stress fibres around the nucleus tend to adopt a straight morphology for large SAs. The quantification of θ could also be used to describe the evolution of R x , such as where l is the long axis of the cell. As shown in Figure 4e , predicted R x values are consistent with those measured from nuclear deformations. Then we assumed that the whole amount of tension per cell is related to the tension generated in actomyosin cables acting on the nucleus. By combining the quantification of T f from TFM experiments ( Fig. 3d ) and the quantification of θ from confocal imaging ( Fig. 4d ), we estimated F c by using equation (1). We found that compressive forces acting on the nucleus of elongated cells (CSI ∼ 0.26) increased with the SA, following a sigmoidal curve ( Fig. 4f ). Interestingly, this finding explains why we observed a rounded nucleus on small SA ( Fig. 2b )—that is, low compressive forces—whereas the nucleus was significantly deformed on large SAs—that is, high compressive forces ( Supplementary Fig. S5 and Supplementary Movies 4 and 5 ). Considering the compression stress, σ = F c / A 0 , and the compression strain, ɛ =Δ R / R 0 (with Δ R = R 0 – R x ), the Young's modulus of the nucleus, E n , is given by: where R 0 is the initial radius of the nucleus and A 0 is the contact area between the nucleus and actin filaments through which the compressive forces are applied. By using experimental values for R 0 and A 0 (see Methods), equation (3) allows us to predict an increase in the nuclear Young's modulus as compressive forces increased ( Fig. 4g ), suggesting a force-dependent stiffening response of the nucleus. By extrapolating the curve shown in Figure 4e , we estimated the nuclear Young's modulus at zero-force condition about E 0 =5.0±0.6 kPa, which is consistent with the nuclear elastic modulus of 5.1±3.0 kPa found by microplate experiments on spread ECs [36] . Nuclear shape remodelling is accompanied by nuclear volume loss To describe the nuclear morphology with more accuracy, we reported the long, a , the short, b , axis and the height, c , of the nucleus quantified by laser scanning confocal microscopy ( Fig. 5a ). When analysing the evolution of the long-to-short axis ratio of the nucleus, a/b , and its projected area as a function of CSI ( Fig. 5b,c ), we found that these two parameters display opposite evolution. Indeed, the nuclear aspect ratio is characterized by a threefold increase as CSI decreases, while the mean projected area of the nucleus was found to decrease by ∼ 22%. To search for the origin of this behaviour, we next assumed an ellipsoidal shape for the nucleus to estimate the volume and the surface area of the nucleus. Surprisingly, we found that the nuclear shape remodelling results in a surface area and volume decrease of ∼ 22 and ∼ 50%, respectively ( Fig. 5d ). This observation could be explained by a shrinkage of the nucleus due to the highly folded structure of the nuclear membrane [37] . Then we investigated the effect of blebbistatin treatment and intermediate filament inhibitors on nuclear volume for circular (CSI ∼ 1) and elongated (CSI ∼ 0.26) ECs. We found that the nuclear volume of circular-shaped cells was not affected by actomyosin inhibition, whereas the nuclear volume of elongated cells was significantly increased with blebbistatin treatment ( Supplementary Fig. S6 ). These results confirm that the nucleus of circular-shaped cells is not altered by tension in actomyosin filaments ( Supplementary Movie 2 ) and are consistent with the evolution of NSI in response to inhibitors, as observed in the Figure 2c . The disruption of intermediate filaments in elongated ECs induced a decrease in the nuclear volume ( Supplementary Fig. S7 ), confirming that intermediate filaments contribute to nuclear shape stability by balancing intracellular forces. Interestingly, the nuclear volume loss that accompanied the overall nuclear remodelling process ( Fig. 5d ) supports the stiffening hypothesis of the nucleus as predicted by our model ( Fig. 4g ), therefore suggesting a deep remodelling of the nuclear architecture in response to cell elongation. 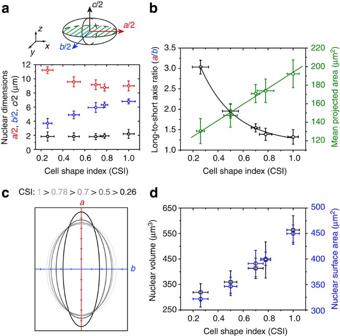Figure 5: The nuclear shape remodelling is accompanied by a nuclear volume loss. (a) Schematic representation of the long axis (a, in red), the short axis (b, in blue), the height (c, in black) and the projected area (dashed green zone) of a nucleus assuming a spheroidal morphology. Quantitative measurements ofa,bandcfor 1,600 μm2shaped cells (1≥CSI≥0.26) were carried out by laser scanning confocal microscopy. The evolution ofa/2 (in red),b/2 (in blue) andc/2 (in black) was plotted as a function of the CSI. Data are given as mean±s.d. with 8≤n≤12. (b) The long-to-short axis ratio (a/b, black curve) and the projected area (green curve), corresponding to the green dashed area in the cartoon presented ina, were plotted as a function of the CSI for SA=1,600 μm2. Data are given as mean±s.d. with 8≤n≤12. (c) Superimposed nuclear outlines show clearly the increase in the long-to-short axis ratio, whereas the nuclear projected area decreases. (d) The nucleus was fitted with an ellipsoidal morphology to calculate the evolution of the nuclear volume (in black) and the nuclear surface area (in blue) versus CSI. During cell elongation, both volume and surface area of the nucleus decrease. Data are given as mean±s.d. with 8≤n≤12. Figure 5: The nuclear shape remodelling is accompanied by a nuclear volume loss. ( a ) Schematic representation of the long axis ( a , in red), the short axis ( b , in blue), the height ( c , in black) and the projected area (dashed green zone) of a nucleus assuming a spheroidal morphology. Quantitative measurements of a , b and c for 1,600 μm 2 shaped cells (1≥CSI≥0.26) were carried out by laser scanning confocal microscopy. The evolution of a /2 (in red), b /2 (in blue) and c /2 (in black) was plotted as a function of the CSI. Data are given as mean±s.d. with 8≤ n ≤12. ( b ) The long-to-short axis ratio ( a / b , black curve) and the projected area (green curve), corresponding to the green dashed area in the cartoon presented in a , were plotted as a function of the CSI for SA=1,600 μm 2 . Data are given as mean±s.d. with 8≤ n ≤12. ( c ) Superimposed nuclear outlines show clearly the increase in the long-to-short axis ratio, whereas the nuclear projected area decreases. ( d ) The nucleus was fitted with an ellipsoidal morphology to calculate the evolution of the nuclear volume (in black) and the nuclear surface area (in blue) versus CSI. During cell elongation, both volume and surface area of the nucleus decrease. Data are given as mean±s.d. with 8≤ n ≤12. Full size image Chromatin condensation and low cell proliferation rate Starting from the above results, an important question that needed to be addressed was therefore whether large-scale changes of cell shape may affect nuclear architecture and functions. To answer this question, we first examined the chromatin organization by using a quantitative procedure based on DAPI staining [38] . Indeed, the uptake of DAPI depends on the total amount of DNA, but also on its level of condensation [39] . For these reasons, the average spatial density corresponding to the ratio between the integrated fluorescence intensity and the volume of the nucleus is a reliable indicator of the in-situ average chromatin condensation. 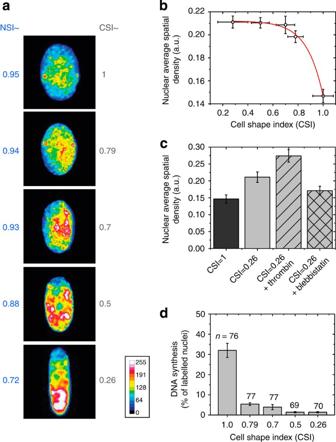Figure 6: Cell elongation leads to chromatin condensation and affects cell proliferation. (a) Successive changes of the level of chromatin condensation as the NSI decreases. Intensities of DNA staining were digitized in 256 bits and colour coded (from high to low: white, purple, red, orange, yellow, green, light blue and dark blue). Highly condensed domains show higher fluorescence intensity with respect to the less condensed ones. (b) Evolution of the mean average spatial density of the nucleus as a function of the CSI. (c) Elongated cells (CSI∼0.26, light grey bar) were treated with thrombin (hatched bar) and blebbistatin (cross-hatched bar). The average spatial density quantified by DAPI staining was compared with circular-shaped cells (dark grey bar). (d) Evolution of the DNA synthesis in response to cell shape changes (1≥CSI≥0.26). Data are given as mean±s.d. withn≥12 forb,cand 69≤n≤76 ford. As shown in Figure 6a , marked reorganization of chromatin distribution was associated with nuclear deformation. Highly condensed chromatin domains show higher fluorescence intensity with respect to the less condensed ones. When cells were disk-shaped, chromatin was largely extended within a rounded nucleus, with few small condensed domains localized centrally. As the cell elongated, the nucleus became deformed and chromatin tended to condense starting from the nuclear periphery towards the centre to become rapidly packaged ( Fig. 6a ). By plotting the nuclear average spatial density as a function of CSI ( Fig. 6b ), we showed that the average spatial density of the nucleus increased with decreasing CSI, establishing that condensation of chromatin takes place as the cell elongates. It is noteworthy that nuclear stiffening ( Fig. 4e ) and chromatin condensation ( Fig. 6b ) in response to cell elongation are both consistent with micropipette aspiration experiments [40] , suggesting that the rheological parameters of the nucleus is largely set by the level of chromatin condensation. As shown in Figure 6c , we observed that thrombin treatment increased the chromatin condensation by ∼ 31%, whereas blebbistatin induced a decrease of ∼ 20%. These results indicate that large nuclear deformations previously observed for thrombin-treated cells are associated with a high level of chromatin compaction and confirm the role of actomyosin filaments in the modulation of the nuclear architecture. We next investigated the effect of large-scale cell shape changes on the cell proliferation rate. The DNA synthesis of ECs, which provides an indication of the cell proliferation rate, was determined by the percentage of 5-bromo-2′-deoxyuridine (BrdU)-positive cells after a cumulative incorporation (8 h labelling). The proliferation rate was found to be drastically affected by cell elongation ( Fig. 6d ). Furthermore, we observed a linear relation between the average spatial density and cell proliferation, suggesting that DNA synthesis could be altered by chromatin condensation ( Supplementary Fig. S8 ). Figure 6: Cell elongation leads to chromatin condensation and affects cell proliferation. ( a ) Successive changes of the level of chromatin condensation as the NSI decreases. Intensities of DNA staining were digitized in 256 bits and colour coded (from high to low: white, purple, red, orange, yellow, green, light blue and dark blue). Highly condensed domains show higher fluorescence intensity with respect to the less condensed ones. ( b ) Evolution of the mean average spatial density of the nucleus as a function of the CSI. ( c ) Elongated cells (CSI ∼ 0.26, light grey bar) were treated with thrombin (hatched bar) and blebbistatin (cross-hatched bar). The average spatial density quantified by DAPI staining was compared with circular-shaped cells (dark grey bar). ( d ) Evolution of the DNA synthesis in response to cell shape changes (1≥CSI≥0.26). Data are given as mean±s.d. with n ≥12 for b , c and 69≤ n ≤76 for d . Full size image Our results show that actin filaments are essential factors in the mechanical process of nuclear remodelling and establish for the first time a distinct function for central and apical actin structures. Our findings support a model of a gradual anisotropic contraction dipole as the cell elongates, whereby lateral compressive forces acting on the nucleus are driven by a coupling of anisotropic tension and central actin filaments distribution. Furthermore, our results show the unrevealed importance of the cell SA in the nuclear shape remodelling process. We devised a simple mechanical model that relates the variations of orientation and tension in central actin filaments to nuclear deformations. This model describes how the extent of cell elongation induces a growing increase of tension in central actomyosin cables that regulate the nuclear shape by applying lateral compressive forces on both sides of the nucleus. Our study, for the time to our knowledge, therefore provides a unifying perspective on the mechanistic regulation between cell and nuclear shape ( Fig. 7 ). 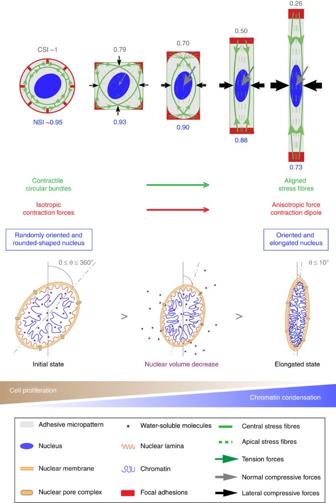Figure 7: Model for the mechanical orchestration between cell and nuclear shape changes. As the cell elongates, the nucleus initially rounded and randomly oriented becomes significantly deformed and oriented with respect to the long-cell axis direction. Cellular elongation is associated with the formation of parallel actin bundles on either sides of the nucleus and the anisotropy of FAs. During cell elongation, tension in actin filaments increases and results in a high level of compressive forces acting laterally on both sides of the nucleus. The magnitude of compressive forces is denoted by the thickness of the black arrows. Changes in nuclear shape induce a loss of nuclear volume, which causes conformational changes in chromatin structure that significantly affect the cell proliferation. Figure 7: Model for the mechanical orchestration between cell and nuclear shape changes. As the cell elongates, the nucleus initially rounded and randomly oriented becomes significantly deformed and oriented with respect to the long-cell axis direction. Cellular elongation is associated with the formation of parallel actin bundles on either sides of the nucleus and the anisotropy of FAs. During cell elongation, tension in actin filaments increases and results in a high level of compressive forces acting laterally on both sides of the nucleus. The magnitude of compressive forces is denoted by the thickness of the black arrows. Changes in nuclear shape induce a loss of nuclear volume, which causes conformational changes in chromatin structure that significantly affect the cell proliferation. Full size image Interestingly, this model not only provides a conceptual framework of the mechanical coupling between cell and nuclear shape but also predicts a stiffening of the nucleus as the cell elongates. We demonstrated that this nuclear stiffening occurs in response to cell elongation due to a significant loss of nuclear volume, which induces chromatin condensation and dramatically affects cell proliferation. Our results give a physical insight in the stiffening of EC nuclei [41] and are consistent with previous works indicating that an important part of the nuclear volume ( ∼ 45%) of isotropic ECs remains virtually free of DNA [42] , and that nuclear pores expand and transport rates increase when cells physically elongate [43] . As the typical timescale of stress fibre assembly (from several minutes to few hours) is larger than the characteristic plastic time of the nucleus ( τ p ∼ 10 s) [40] , our model is also consistent with the current rheological view of the nucleus, which considers that the nucleus is stiff and resists distortions at short times, but it softens and deforms more readily at longer times [40] , [44] . Additional investigations using computational models [45] to include fluid leakage through the pores and the relative contribution of the nuclear envelope could be useful to elucidate the underlying mechanisms of this cytoskeleton-mediated hardening of the nucleus. In addition, given recent interests on molecular linkages between apical actin filaments and nuclear membrane [18] , [19] , it will be interesting to investigate whether such links exist for central actin filaments and influence the force transmission process. Stamp fabrication and microcontact printing Micropatterns of various shapes (circles, squares and rectangles with aspect ratios of 1:2, 1:4 and 1:10) and various areas (600, 800, 1,200, 1,600, 2,000 μm 2 ) were generated to a silicon master by deep reactive-ion etching (FH Vorarlberg University of Applied Sciences, Microtechnology, Dornbirn, Austria) from a chromium photomask (Toppan Photomask, Corbeil Essonnes, France). The silicon surface was passivated with a fluorosilane (tridecafluoro-1,1,2,2-tetrahydrooctyl-1-trichlorosilane, Gelest) for 30 min, and microstamps were obtained by molding the silanized silicon master with polydimethylsiloxane, PDMS, (Sylgard 184 Silicone Elastomer Kit; Dow Corning, Midland, MI) cured for 4 h at 60 °C. PDMS stamps were oxidized in an ultraviolet/O 3 oven for 8 min and inked with a 25 μg ml −1 FN solution from human plasma (Sigma, St Louis, MO) for 1 h at room temperature. Then PDMS stamps were dried under filtered air and gently pressed onto a flat PDMS-coated glass coverslip. Uncoated regions were blocked by incubating for 5 min in a 1% Pluronic F-127 solution [46] (BASF, Mount Olive, NJ) and washed three times in PBS. Cell culture and immunocytochemistry Primary human umbilical vein endothelial cells (Cells Applications, San Diego, CA) were grown in complete endothelial cell growth medium (Cells Applications) supplemented with 1% antibiotics and antimycotics (PAA Laboratories, Pasching, Austria) and maintained at 37 °C in a humidified atmosphere with 5% CO 2 . Human umbilical vein endothelial cells, used between passages 2 and 8, were deposited on microprinted coverslips at a concentration of about 15,000 cells ml −1 . After 24 h, cells were permeabilized with a solution of 4% paraformaldehyde (Electron Microscopy Sciences, Hatfield, PA), fixed with 0.05% Triton X-100 (Sigma) in PBS (PAA Laboratories) for 15 min at 37 °C and washed three times in PBS. Cells were incubated for 45 min at 37 °C with 4,6-diamidino-2-phenylindole dihydrochloride (Molecular Probes, Invitrogen, Cergy Pontoise, France), Alexa Fluor 488 Phalloidin (Molecular Probes, Invitrogen) and monoclonal anti-vinculin antibody produced in mouse (HVIN-1 clone, Sigma), washed three times in PBS, and incubated for 45 min at 37 °C with a goat anti-mouse antibody labelled with tetramethylrhodamine (Molecular Probes, Invitrogen). Slides were mounted in Slow Fade Gold Antifade (Molecular Probes, Invitrogen). Pharmacological treatments Specific pharmacological agents were used to inhibit the polymerization of actin filaments [47] (latrunculin-A, Enzo Life Sciences, Zandhoven, Belgium), microtubules [48] (Colchicine, Enzo Life Sciences) and to collapse the intermediate filament network [49] , [50] (Acrylamide and Calyculin A, Sigma). Blebbistatin (Enzo Life Sciences) was used to inhibit myosin II contractility [51] . Cells grown on 1,600 μm 2 FN islands were treated separately for 1 h with latrunculin-A at 1 μM in dimethylsulphoxide, DMSO (Sigma), colchicine at 10 μM in sterile water, acrylamide at 40 mM in sterile water, blebbistatin at 100 μM in DMSO and for 15 min with calyculin A at 2.5 nM in ethanol. A stock solution of thrombin (Sigma) was obtained by dilution in a 0.1% bovine serum albumin solution (PAA Laboratories) and thrombin was used at a concentration of 1 U ml −1 for 5 min. Control experiments showed that DMSO up to 0.5% does not affect ECs, and additional experiments demonstrated that the effects of all of these pharmacological agents were sustained for the entire experimental period. DIC, epifluorescence and confocal imaging Fixed and immunofluorescence-stained preparations were observed in DIC, epifluorescence and confocal mode with a Nikon Eclipse Ti-E motorized inverted microscope (Nikon C1 scanhead; Nikon, Japan) equipped with ×40 DIC, ×40 Plan Apo (NA 1.45, oil immersion), ×60 Plan Apo (NA 1.45, oil immersion) and ×100 Plan Apo (NA 1.45, oil immersion) objectives, two lasers (Ar ion 488 nm; HeNe, 543 nm) and a modulable diode (408 nm). DIC and epifluorescence images were captured with a Roper QuantEM:512SC EMCCD camera (Photometrics, Tucson, AZ) using Capture-Pro software (Photometrics). Confocal images were acquired with NIS Elements Advanced Research 3.0 software (Nikon) by using small Z-depth increments between focal sections (0.15 μm) and then analysed with a combination of NIS Elements AR and ImageJ [52] softwares. Confocal frames were systematically deconvoluted using an AutoQuant module of NIS Elements AR Software based on an Iterative Blind Deconvolution algorithm [53] . As the quality of the deconvolution process depends on the number of iterations, we determined a number of 15 iterations on visual inspection of the resulting image. Cell and nuclear shape analysis To quantify the variation in nuclear shape, we extracted the contour of individual stained nucleus with a custom-written MATLAB software that automatically segmented images of fluorescent nuclei and traced the best-fitted outline ellipse to determine long, a, and short, b, axis, perimeter and projected area of each nucleus. To quantify the nuclear orientation, the orientation of the best-fitted ellipse was calculated with respect to the long cell axis for rectangular-shaped cells (0.70≤CSI≤0.26) and to the vertical axis of circular (CSI ∼ 1) and square-shaped cells (CSI ∼ 0.79). Areas and perimeters of shaped-cells were measured by ImageJ on DIC images and used to calculate the CSI from the relationship: CSI=4π×area/(perimeter) [2] . The CSI assumes values between one (circular shape) and zero (elongated, linear morphology). A similar relationship was used to calculate the NSI from the nuclear projected area and the nuclear perimeter. Experimental values of the contact area between the nucleus and lateral actin filaments, A 0 , were determined on elongated ECs (CSI ∼ 0.26) stained for nuclear DNA (DAPI) and actin (Alexa Fluor 488 Phalloidin). Confocal scanning Z-stacks were deconvoluted to display three-dimensional volume rendering to determine the mean width of central actin cables from a side view and the mean contact length between lateral actin fibres and nuclei from a normal view. Assuming a rectangular shape, the contact area was then estimated for each SA (from 600 to 2,000 μm 2 ). By assuming an ellipsoidal shape, the volume, V n , and the surface area, A n , of the nucleus were calculated from quantitative measurements of the nuclear dimensions performed by confocal microscopy. The nuclear volume, V n , was obtained from the following formula: whereas the nuclear surface area, A n , was estimated from the following approximate formula: where 2 a , 2 b and 2 c correspond to the length, the width and the height of the nucleus, respectively, with p= 1.6075. Traction force microscopy data measurement and analysis Polyacrylamide gels (0.1% bis and 5% acrylamide; 70 μm thick) containing 1:50 volume of carboxylate-modified fluorescence latex beads (0.2 μm Fluospheres, Molecular Probes, Eugene, OR) were fabricated on 25-mm diameter glass coverslips. The Young's modulus of the gel was estimated to be 9 kPa using Dynamic Mechanical Analysis (Mettler Toledo, Switzerland). FN-coated PDMS stamps were allowed to react with the activated gel for 1 h at 37 °C to create FN-coated adhesive islands. After removal of the excess of FN by washing with PBS, unprinted areas of the gels were passivated with a bovine serum albumin solution overnight. Fluorescence images of the gel containing fluorescent beads immediately beneath the patterned cells were taken during the cell detachment. The change of the position of the fluorescence beads were measured in Matlab software using an algorithm described previously [54] . This yielded the discretized displacement field between two consecutive frames. The calculated displacements were summed up to determine the overall two-dimensional displacement field. The traction field was then calculated from the displacement field by adapting the algorithm previously developed [35] . This algorithm solved the inverse of the Boussinesq solution from the displacement field on the surface of an elastic halfspace to obtain the traction field when the mechanical properties of the gel are known. The Poisson ratio of the gel was assumed to be close to 0.5 (ref. 55 ). The interior of the cell was subdivided into 64 μm 2 squares to approximate the discretized localization of contractile forces. Apparent chromatin condensation and DNA synthesis Spatial chromatin organization was visualized by staining with DAPI, a fluorescent dye that selectively binds to the double-stranded DNA. After permeabilization in 0.05% Triton X-100 solution (Sigma), ECs were stained with 25 μg ml −1 DAPI and a stack of nuclear images at different focal positions along the z axis (0.15 μm intervals) were acquired in confocal scanning microscopy. To obtain quantitative information, shading correction and dark image substraction were applied in MATLAB to each image [38] and a constrained deconvolution in NIS Elements AR software was used to sharpen the image [56] . After normalizing for time exposure, the integrated fluorescence intensity was calculated as the sum of the intensity of each pixel. The total fluorescence intensity was then divided by the nuclear volume to obtain the average spatial density, which correlates with the average chromatin packing ratio [56] , [57] , and as such is indicative of chromatin condensation. The proliferative activity in shape-engineered ECs has been investigated by detecting the incorporation of BrdU into cellular DNA. BrdU is a thymidine analogue that incorporates into the DNA-synthetizing nuclei, which can be identified immunohistochemically using an anti-BrdU monoclonal antibody. BrdU cumulative labelling was carried out with injection of 10 μM BrdU in PBS from t =16 h to 24 h, with intervals of 2 h. After cumulative BrdU injections, cells were fixed in paraformaldehyde and DNA was denatured in DNase I (Sigma) at 62.5 U ml −1 for 30 min at 37 °C. How to cite this article: Versaevel, M. et al . Spatial coordination between cell and nuclear shape within micropatterned endothelial cells. Nat. Commun. 3:671 doi: 10.1038/ncomms1668 (2012).